Microcephaly disease geneWdr62regulates mitotic progression of embryonic neural stem cells and brain size Human genetic studies have established a link between a class of centrosome proteins and microcephaly. Current studies of microcephaly focus on defective centrosome/spindle orientation. Mutations in WDR62 are associated with microcephaly and other cortical abnormalities in humans. Here we create a mouse model of Wdr62 deficiency and find that the mice exhibit reduced brain size due to decreased neural progenitor cells (NPCs). Wdr62 depleted cells show spindle instability, spindle assembly checkpoint (SAC) activation, mitotic arrest and cell death. Mechanistically, Wdr62 associates and genetically interacts with Aurora A to regulate spindle formation, mitotic progression and brain size. Our results suggest that Wdr62 interacts with Aurora A to control mitotic progression, and loss of these interactions leads to mitotic delay and cell death of NPCs, which could be a potential cause of human microcephaly. Neural progenitor cells (NPCs) of the embryonic neocortex initially comprise a large population of the neuroepithelial cells and, as development proceeds, radial glia located in the ventricular zone (VZ) continue to provide a source of NPCs. Radial glia undergo symmetric cell divisions to replenish themselves and asymmetric divisions to produce postmitotic neurons or intermediate neural progenitors (INPs) [1] . Harnessing the potential of NPCs holds promise for the treatment of neuronal injury and neurodegenerative diseases, and dysfunction of NPCs is at the root of numerous neurological disorders [2] , [3] . However, the in vivo regulatory mechanisms that control NPC self-renewal and differentiation are incompletely defined. One approach for investigating the regulatory mechanisms underlying NPC biology is through the study of animal models of human neurological disorders. Autosomal recessive primary microcephaly (MCPH) is a congenital brain disorder characterized by a small brain size without severe effects on brain structure [4] , [5] . Human genetic studies have identified ten MCPH loci, and most MCPH proteins localize to the centrosome or spindle pole for at least part of the cell cycle. These MCPH proteins have been implicated in different biological processes from centriole biogenesis, centrosome maturation, spindle position, gene regulation, to DNA repair among others [4] , [5] , [6] , [7] . However, due to limited numbers of MCPH animal models, it remains unclear as to what kinds of cellular processes are disrupted by MCPH gene mutations that result in microcephaly, what are the molecular mechanisms regulating these cellular processes, and how these regulatory mechanisms underlie NPC biology. Although the aetiology of microcephaly remains unclear, the predominant model is that disruptions in spindle orientation result in altered symmetric/asymmetric cell division of the NPCs, leading to depletion of NPCs and promotion of neuronal differentiation. However, impaired spindle orientation and altered symmetric division are not sufficient to cause MCPH [4] , [5] , as neurogenesis and brain size appear normal in mice mutant for the polarity determinant aPKCλ, which is essential for symmetric cell division control [8] or following depletion of LGN, a non-centrosomal determinant of spindle orientation and symmetric cell division [9] . Therefore, it remains unclear as to what cellular processes are disrupted due to microcephaly gene mutations, and to what extent and how these defective cellular behaviours contribute to the microcephaly phenotypes. Wdr62 ( MCPH2; OMIM 604317 ) is the second most common genetic cause of microcephaly, and mutations in human WDR62 result in microcephaly and a wide spectrum of additional cortical abnormalities including heterotopia, lissencephaly, polymicrogyria and schizencephaly [10] , [11] , [12] . However, the in vivo functions and the mechanisms of Wdr62 action during normal cortical development remain unclear. Here we show that the loss of Wdr62 functions in mice results in mitotic delay and cell death of NPCs, which leads to reduced brain size. Wdr62 depleted cells exhibit altered spindle stability, spindle assembly checkpoint (SAC) activation, delayed mitotic progression, and cell death. Mechanistically, Wdr62 associates and genetically interacts with the spindle assembly factor Aurora A to control NPC mitosis and brain size. Together, our studies define Wdr62 as an essential regulator of embryonic NPC mitotic progression, and suggest that the delay of mitotic progression and cell death could be potential causes of human microcephaly. Wdr62 deficiency results in dwarfism and microcephaly in mice To investigate the molecular mechanisms underlying Wdr62 function, we created a mouse model using gene-trap ES cells in which the Wdr62 gene has been disrupted by the insertion of a β-geo reporter. Wdr62 is comprised of 15 WD-repeat domains ( Fig. 1a ). The insertion site mapped to the intronic region between exons 14 and 15 of Wdr62 ( Fig. 1a ). Western blot analyses using a C-terminal specific antibody that we generated showed a significant reduction of Wdr62 protein in homozygous mutant embryos ( Fig. 1b,c ). The presence of some normal length Wdr62 detected with the C-terminal antibody in the homozygous mutant indicates this is a hypomorphic allele, likely due to occasional normal splicing and skipping of the gene-trap vector. 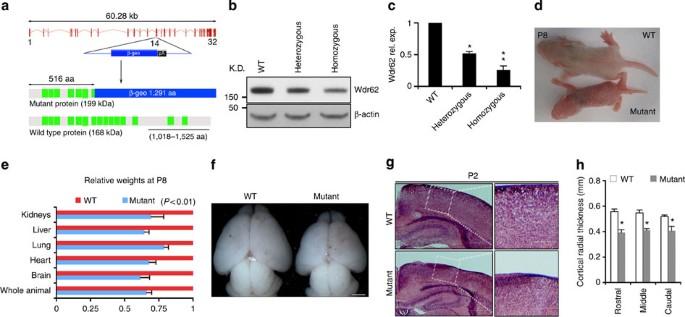Figure 1:Wdr62deficient mice exhibit dwarfism and microcephaly. (a) Genomic structure ofWdr62locus on mouse chromosome 7; black line represents the protein region (1,018–1,525 aa) used for antibody generation. (b) Western blot analyses of Wdr62 protein expression in cerebral cortex of E15.5 wild-type (WT), heterozygous and homozygous mutant embryos using the C-terminal Wdr62 antibody. The presence of some normal length Wdr62 detected with the C-terminal antibody in the homozygous mutant indicates that this allele is hypomorphic, likely due to occasional skipping of the gene-trap vector. β-actin as loading control. (c) Quantification of Wdr62 protein expression from experiments similar tob. Mean±s.e.m. of data from three separate experiments in which two embryos per group are included for each experiment (*P<0.05, **P<0.01, student’st-test). rel., relative; exp., expression. (d)Wdr62mutant and its WT littermate on postnatal day 8 (P8). (e) Relative weights of different organs from P8 wild-type and mutant mice. Mean±s.e.m. of data from five separate experiments (P<0.01, Student’st-test). (f) Dorsal views of P2 WT and mutant mouse brains. Scale bar, 1 mm. (g) Coronal sections of P2 cerebral cortex stained with haematoxylin and eosin. Scale bar, 0.5 mm in left panels; 0.2 mm in enlarged right panels. (h) TheWdr62deficient cortex shows a decreased radial thickness in all regions. All data represent mean±s.e.m. of three independent experiments (two embryos per group per experiment; *P<0.05, Student’st-test). Figure 1: Wdr62 deficient mice exhibit dwarfism and microcephaly. ( a ) Genomic structure of Wdr62 locus on mouse chromosome 7; black line represents the protein region (1,018–1,525 aa) used for antibody generation. ( b ) Western blot analyses of Wdr62 protein expression in cerebral cortex of E15.5 wild-type (WT), heterozygous and homozygous mutant embryos using the C-terminal Wdr62 antibody. The presence of some normal length Wdr62 detected with the C-terminal antibody in the homozygous mutant indicates that this allele is hypomorphic, likely due to occasional skipping of the gene-trap vector. β-actin as loading control. ( c ) Quantification of Wdr62 protein expression from experiments similar to b . Mean±s.e.m. of data from three separate experiments in which two embryos per group are included for each experiment (* P <0.05, ** P <0.01, student’s t -test). rel., relative; exp., expression. ( d ) Wdr62 mutant and its WT littermate on postnatal day 8 (P8). ( e ) Relative weights of different organs from P8 wild-type and mutant mice. Mean±s.e.m. of data from five separate experiments ( P <0.01, Student’s t -test). ( f ) Dorsal views of P2 WT and mutant mouse brains. Scale bar, 1 mm. ( g ) Coronal sections of P2 cerebral cortex stained with haematoxylin and eosin. Scale bar, 0.5 mm in left panels; 0.2 mm in enlarged right panels. ( h ) The Wdr62 deficient cortex shows a decreased radial thickness in all regions. All data represent mean±s.e.m. of three independent experiments (two embryos per group per experiment; * P <0.05, Student’s t -test). Full size image Wdr62 heterozygous mice were viable and fertile with normal size. Homozygous mutant mice showed dwarfism at birth, and their body and organ size remained smaller than littermates throughout adulthood ( Supplementary Fig. 1 ). Homozygous mutants have a normal lifespan but fertility is reduced. In postnatal day 8 mutants, organ mass was decreased in relative proportion to total body weight ( Fig. 1d,e ). Brain size was also reduced at P2 and P8 with a general 20% reduction in the thickness of the cortex in mutant Wdr62 brains compared with littermates ( Fig. 1f–h ). This relatively proportional dwarfism in the mouse model versus selective brain reduction in human patients may be expected as the encephalization quotient for human is 7.4–7.8 whereas for mouse it is 0.5 (ref. 13 ), and the relative ratio of cortex surface between human and mouse is 1,000:1 (ref. 14 ). Mutant embryos showed growth retardation at embryonic day 17.5 (E17.5) but there was no morphological difference at E15.5. Our studies suggest that Wdr62 is critically required for murine growth control. Wdr62 loss leads to depletion of cortical neural progenitors To determine the role of Wdr62 in brain formation and the mechanism underlying microcephaly, we examined the cerebral cortex during embryogenesis and early postnatal development. Thinning of the cerebral cortex was detected in E17.5 embryos and was more pronounced in P2 mutant brains but there was no significant difference in cerebral cortex size at E15.5 ( Fig. 2a–c,e,f ). Staining of cortical layer markers, including Tbr1 and Ctip2 (layers V–VI) and Cux1 (layers II–IV), showed a reduction of neurons in layers II–VI of the P2 mutant cerebral cortex, with the most pronounced thinning of the later-born superficial cortical layers (for example, Cux1 positive neurons) relative to the early-born deeper layers ( Fig. 2a,b ). 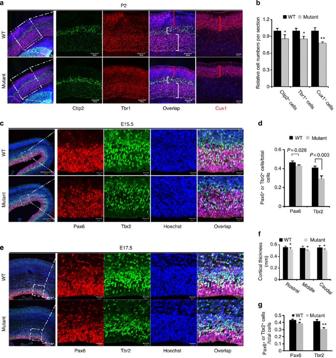Figure 2:Wdr62deficiency results in thinning of cortical layers and depletion of cortical NSCs and INPs. (a) Confocal microscope images of coronal sections from P2 wild-type (WT) and mutant cortex stained with antibodies against Ctip2 (green), Tbr1 (red) and Cux1 (red). Hoechst stains nuclei (blue). Right panels are enlargements of the regions outlined by white dotted boxes. White brackets highlight the layer V–VI labelled by Ctip2 and Tbr1, respectively. Red brackets highlight layer II–IV labelled by Cux. Scale bar, 100 μm. (b) Quantification of relative Ctip2−, Tbr1− and Cux1-positive cells per section. All data represent mean±s.e.m. of three independent experiments (two embryos per group per experiment; *P<0.05, **P<0.01, Student’st-test). (c,e) Confocal micrographs of coronal sections from E15.5 (c) or E17.5 (e) wild-type and mutant cortex stained with antibodies against Pax6 (red), Tbr2 (green). Hoechst stains nuclei (blue). Right panels are enlargements of white dotted box regions. Scale bar, 200 μm (left panels); 20 μm (right panels). (d,g) Quantification of percentage of Pax6- or Tbr2-positive cells per total number of cells within a 2.57 × 104μm2field in experimentcor a 2.96 × 104μm2field in experimenteas indicated by white dotted boxes. All data represent mean±s.e.m. of three independent experiments (two embryos per group per experiment). Ind,P=0.026 (Pax6), 0.003 (Tbr2), and ing, *P=0.015 (Pax6), **P=0.003 (Tbr2). Student’st-test was carried out for statistical analyses. (f) TheWdr62deficient cortex shows a decreased radial thickness in all regions at E17.5. All data represent mean±s.e.m. of three independent experiments (two embryos per group per experiment; *P<0.05, Student’st-test). Figure 2: Wdr62 deficiency results in thinning of cortical layers and depletion of cortical NSCs and INPs. ( a ) Confocal microscope images of coronal sections from P2 wild-type (WT) and mutant cortex stained with antibodies against Ctip2 (green), Tbr1 (red) and Cux1 (red). Hoechst stains nuclei (blue). Right panels are enlargements of the regions outlined by white dotted boxes. White brackets highlight the layer V–VI labelled by Ctip2 and Tbr1, respectively. Red brackets highlight layer II–IV labelled by Cux. Scale bar, 100 μm. ( b ) Quantification of relative Ctip2−, Tbr1− and Cux1-positive cells per section. All data represent mean±s.e.m. of three independent experiments (two embryos per group per experiment; * P <0.05, ** P <0.01, Student’s t -test). ( c , e ) Confocal micrographs of coronal sections from E15.5 ( c ) or E17.5 ( e ) wild-type and mutant cortex stained with antibodies against Pax6 (red), Tbr2 (green). Hoechst stains nuclei (blue). Right panels are enlargements of white dotted box regions. Scale bar, 200 μm (left panels); 20 μm (right panels). ( d , g ) Quantification of percentage of Pax6- or Tbr2-positive cells per total number of cells within a 2.57 × 10 4 μm 2 field in experiment c or a 2.96 × 10 4 μm 2 field in experiment e as indicated by white dotted boxes. All data represent mean±s.e.m. of three independent experiments (two embryos per group per experiment). In d , P =0.026 (Pax6), 0.003 (Tbr2), and in g , * P =0.015 (Pax6), ** P =0.003 (Tbr2). Student’s t -test was carried out for statistical analyses. ( f ) The Wdr62 deficient cortex shows a decreased radial thickness in all regions at E17.5. All data represent mean±s.e.m. of three independent experiments (two embryos per group per experiment; * P <0.05, Student’s t -test). Full size image To guide our mechanistic studies, we assessed the distribution of Wdr62 RNA and protein in mouse E15.5 cerebral cortex two days before cortical thinning was detected in the mutant embryos. These experiments showed broad expression of Wdr62 in both the VZ/subventricular zone and cortical plate ( Supplementary Fig. 2a–g ). Ventricular expression of Wdr62 correlated with Nestin-positive NPCs ( Supplementary Fig. 2d,e ). Wdr62 expression in the cortical plate and marginal zone (MZ) was detected in postmitotic neurons, coincident with neuron-specific MAP2(a,b) ( Supplementary Fig. 2f,g ). Co-immunolabeling with markers of neural stem cells (NSCs, Pax6) or NPCs (Nestin) indicated that Wdr62 is localized to the cytoplasm in NPCs ( Supplementary Fig. 2h,i ). In differentiated cortical neurons, Wdr62 is prominent in the cytoplasm ( Supplementary Fig. 2j,k ), and is barely detected in Tau1 labelled axons ( Supplementary Fig. 2k ). Immunoblots of whole-cell extracts of cortices from different embryonic stages indicates that Wdr62 expression increases as brain development progresses ( Supplementary Fig. 2l ). Thus, our data are consistent with previous reports [10] , [11] that Wdr62 expression occurs in NPCs as well as postmitotic neurons. To assess whether the reduced number of neurons in the Wdr62 mutant cortex could be due to fewer numbers of NPCs, we examined NSCs and INPs using Pax6 and Tbr2, respectively, in comparable cerebral cortex sections from E15.5 and E17.5 wild-type and morphologically similar mutant littermates. At both E15.5 and E17.5, the numbers of Pax6-positive NSCs and Tbr2-positive INPs were significantly decreased in the mutants ( Fig. 2c–e,g ). Together, these data indicate that Wdr62 is required for the maintenance of NSC and INP populations. Reductions in these progenitor populations, which generate cortical neurons [1] , could then lead to the thinning of the cerebral cortex during prenatal and postnatal brain development. Mitotic arrest and cell death of NPCs in Wdr62 mutants Reduced NSCs and INPs could be due to decreased cell proliferation and/or premature differentiation of NPCs. Bromodeoxyuridine (BrdU) labelling showed slightly decreased number of BrdU-positive cells at E17.5 but no significant difference at E15.5 in the mutant cerebral cortex compared with wild type ( Supplementary Fig. 3a–c ). Tbr2-positive INPs at S phase or M phase were not significantly changed in mutant brains compared with wild type at E15.5 ( Supplementary Fig. 3f–h,j ). Furthermore, mutant NPCs do not appear to differentiate prematurely, as revealed by similar fractions of BrdU + /Ki67 − cells as well as similar spatial distribution of neuronal differentiation markers including TuJ1, Neurofilament and Dcx1 in the mutant cortex compared with wild type ( Supplementary Fig. 4 ). These data suggest that reduced numbers of NPCs in the mutant cortex are not due to a decrease in proliferation rate or premature differentiation. Wdr62 is localized at the centrosome in HeLa cells in interphase, as revealed by co-staining with γ-tubulin, and at the spindle poles during mitotic (M) phase ( Supplementary Fig. 5 ). Depletion of centrosome proteins can lead to mitotic arrest and microcephaly in mice [15] , [16] . To examine whether the reduction in NPCs in mutant brains resulted from dysregulated mitosis, we labelled mitotic cells with phospho-histone H3 (p-H3) antibody and NSCs with Pax6. In E15.5 and E17.5 cerebral cortex, p-H3-positive cells were mainly detected in the VZ/subventricular zone in both wild-type and mutants but the number of p-H3-positive cells was increased in Wdr62 mutant brains ( Fig. 3a–c ). There was a significant increase of p-H3/Pax6 double positive cells, which were mostly in prometaphase/metaphase, in the mutant cortex compared with wild type ( Fig. 3d–g ), suggesting that NSCs/INPs are arrested in the M phase of the cell cycle. Mitotic arrest can induce cell death [17] , [18] . Therefore we assessed cell death by TUNEL staining of comparable coronal sections through wild-type and mutant cerebral cortex at E15.5 and E17.5. This showed significantly increased cell death of NSCs and INPs, but not of differentiated neurons, in mutant brains ( Fig. 3h–k ). Together, these studies indicate that the reduction of NPCs in the mutant cerebral cortex could be due to mitotic arrest of these populations and loss by cell death. 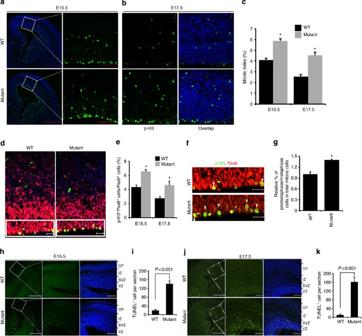Figure 3: Mitotic arrest and cell death inWdr62deficient cerebral cortex. (a,b) Confocal micrographs of coronal sections from E15.5 (a) or E17.5 (b) wild-type and mutant cortex stained with antibodies against phospho-histone H3 (p-H3). Hoechst stains nuclei (blue). Right panels are enlargements of regions outlined by white dotted boxes in left panel. Scale bar, 500 μm (left panels); 100 μm (right panels). (c) Quantification of percentage of p-H3-positive cells per total number of cells within a 1.153 × 105μm2field in experimentaor a 9.750 × 104μm2field in experimentb. All data represent mean±s.e.m. of three independent experiments using two embryos per group per experiment (*P<0.01, Student’st-test). (d) Confocal micrographs of coronal sections from E15.5 wild-type and mutant cortex stained with antibodies against p-H3 (green) and Pax6 (red). Scale bar, 20 μm. (e) Quantification of percentage of p-H3/Pax6 double positive cells per total number of Pax6 positive cells in experimentd. All data represent mean±s.e.m. of three independent experiments using two embryos per group per experiment (*P<0.01, Student’st-test). (f) Confocal micrographs of enlargements of regions outlined by white boxes ind. White arrowheads point to pre-anaphase cells. (g) Quantification of relative percentage of prometaphase or metaphase cells out of the total mitotic cells in the ventricular zone. All data represent mean±s.e.m. of three independent experiments (two embryos per group per experiment; *P<0.01, Student’st-test). (h,j) TUNEL staining (green) on coronal sections of E15.5 (h) or E17.5 (j) cortex revealed significantly higher number of apoptotic cells in mutant compared with wild type. Hoechst stains nuclei (blue). Right panels are enlargements of regions outlined by white dotted boxes. VZ, ventricular zone; SVZ, subventricular zone; IZ, intermediate zone; CP, cortical plate. Scale bar, 500 μm (left panel); 100 μm (middle and right panels). (i,k) Quantification of TUNEL-positive cells from experiments as inhandj, respectively. TUNEL-positive cells were calculated in the entire section. All data represent mean±s.e.m. of three independent experiments (two embryos per group per experiment;P<0.001, Student’st-test). Figure 3: Mitotic arrest and cell death in Wdr62 deficient cerebral cortex. ( a , b ) Confocal micrographs of coronal sections from E15.5 ( a ) or E17.5 ( b ) wild-type and mutant cortex stained with antibodies against phospho-histone H3 (p-H3). Hoechst stains nuclei (blue). Right panels are enlargements of regions outlined by white dotted boxes in left panel. Scale bar, 500 μm (left panels); 100 μm (right panels). ( c ) Quantification of percentage of p-H3-positive cells per total number of cells within a 1.153 × 10 5 μm 2 field in experiment a or a 9.750 × 10 4 μm 2 field in experiment b . All data represent mean±s.e.m. of three independent experiments using two embryos per group per experiment (* P <0.01, Student’s t -test). ( d ) Confocal micrographs of coronal sections from E15.5 wild-type and mutant cortex stained with antibodies against p-H3 (green) and Pax6 (red). Scale bar, 20 μm. ( e ) Quantification of percentage of p-H3/Pax6 double positive cells per total number of Pax6 positive cells in experiment d . All data represent mean±s.e.m. of three independent experiments using two embryos per group per experiment (* P <0.01, Student’s t -test). ( f ) Confocal micrographs of enlargements of regions outlined by white boxes in d . White arrowheads point to pre-anaphase cells. ( g ) Quantification of relative percentage of prometaphase or metaphase cells out of the total mitotic cells in the ventricular zone. All data represent mean±s.e.m. of three independent experiments (two embryos per group per experiment; * P <0.01, Student’s t -test). ( h , j ) TUNEL staining (green) on coronal sections of E15.5 ( h ) or E17.5 ( j ) cortex revealed significantly higher number of apoptotic cells in mutant compared with wild type. Hoechst stains nuclei (blue). Right panels are enlargements of regions outlined by white dotted boxes. VZ, ventricular zone; SVZ, subventricular zone; IZ, intermediate zone; CP, cortical plate. Scale bar, 500 μm (left panel); 100 μm (middle and right panels). ( i , k ) Quantification of TUNEL-positive cells from experiments as in h and j , respectively. TUNEL-positive cells were calculated in the entire section. All data represent mean±s.e.m. of three independent experiments (two embryos per group per experiment; P <0.001, Student’s t -test). Full size image Wdr62 depleted cells exhibit mitotic delay and cell death To probe the cellular roles and functional mechanisms for Wdr62 in mitotic regulation, we turned to mouse embryonic fibroblasts (MEFs). Consistent with our in vivo analyses, there was a significant increase in the number of Wdr62 mutant cells arrested in mitosis, mainly in prometaphase and metaphase ( Fig. 4a,b ). Fluorescence-activated cell sorting to determine DNA content showed a significant increase in 4N DNA content in mutant MEFs ( Fig. 4c,d ). There was also an increase in the sub-G0 (less than 2N) population in the mutant MEFs ( Fig. 4c,e ), suggestive of cell death (black arrowhead in Fig. 4c ). These analyses from MEFs are consistent with the in vivo study ( Fig. 3 ), and suggest that depletion of Wdr62 results in mitotic arrest and cell death. 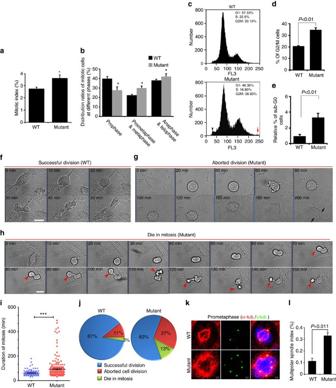Figure 4:Wdr62depleted cells exhibit a delay in mitotic progression and cell death. (a,b) Wild-type (WT) and mutant MEFs at passage 4 were fixed, stained for p-H3 and scored for the frequencies in mitosis (a) and in different mitotic phases as indicated based on nuclear morphology (b). S.e.m. of three independent experiments, counting more than 5,000 cells per experiment (*P<0.05, Student’st-test). (c) Wild-type and mutant MEFs at passage 4 were fixed and stained with propidium iodide, and cell cycle distribution analysed by flow cytometry. In mutant, black arrowhead indicates a significant increase in the sub-G0 (less than 2N) population of mutant MEFs. (d,e) Statistical analysis of results from experimentc. Three independent experiments with MEFs isolated from different embryos were performed; the G2M population (d) and sub-G0 population (e) are significantly increased in mutant cells compared with control (P<0.01, Student’st-test). (f–h) Still images from time-lapse movies of wild-type and mutant MEFs showing successful division (f, wild type), aborted division (g, mutant), delayed mitotic progression and cell death during mitosis (h, mutant). Images were taken every 10 min. Black arrows indicate cell with two nuclei following aborted division. Red arrowheads point to one of the two mutant daughter cells that underwent cell death during mitosis. Scale bar, 20 μm. (i) Quantification of the mitotic duration of wild-type and mutant cells with successful division from experiments as inf–h. Data are expressed as mean±s.d. in seven independent experiments, counting 107 (wild-type) and 235 (mutant) mitotic cells (***P<0.001, Student’st-test test). (j) Statistical analyses of individual cell fates from time-lapse imaging of wild-type and mutant MEFs as in experimentsf–h. Note the significant increase in aborted cell division (red) and cell death in mitosis (green) in mutant compared with WT. (k) Confocal microscope images of MEFs in prometaphase stained with antibodies against α-tubulin (α-tub., red) and γ-tubulin (γ-tub., green). Hoechst stains chromosomes (blue). Note the increased centrosome numbers (γ-tubulin staining) in the mutant compared with WT. Scale bar, 2 μm. (i) Quantification of multipolar spindles in experimentk. Data represents s.e.m. of three independent experiments, counting at least 5,000 MEFs per experiment (P=0.011, Student’st-test). Figure 4: Wdr62 depleted cells exhibit a delay in mitotic progression and cell death. ( a , b ) Wild-type (WT) and mutant MEFs at passage 4 were fixed, stained for p-H3 and scored for the frequencies in mitosis ( a ) and in different mitotic phases as indicated based on nuclear morphology ( b ). S.e.m. of three independent experiments, counting more than 5,000 cells per experiment (* P <0.05, Student’s t -test). ( c ) Wild-type and mutant MEFs at passage 4 were fixed and stained with propidium iodide, and cell cycle distribution analysed by flow cytometry. In mutant, black arrowhead indicates a significant increase in the sub-G0 (less than 2N) population of mutant MEFs. ( d , e ) Statistical analysis of results from experiment c . Three independent experiments with MEFs isolated from different embryos were performed; the G2M population ( d ) and sub-G0 population ( e ) are significantly increased in mutant cells compared with control ( P <0.01, Student’s t -test). ( f – h ) Still images from time-lapse movies of wild-type and mutant MEFs showing successful division ( f , wild type), aborted division ( g , mutant), delayed mitotic progression and cell death during mitosis ( h , mutant). Images were taken every 10 min. Black arrows indicate cell with two nuclei following aborted division. Red arrowheads point to one of the two mutant daughter cells that underwent cell death during mitosis. Scale bar, 20 μm. ( i ) Quantification of the mitotic duration of wild-type and mutant cells with successful division from experiments as in f – h . Data are expressed as mean±s.d. in seven independent experiments, counting 107 (wild-type) and 235 (mutant) mitotic cells (*** P <0.001, Student’s t -test test). ( j ) Statistical analyses of individual cell fates from time-lapse imaging of wild-type and mutant MEFs as in experiments f – h . Note the significant increase in aborted cell division (red) and cell death in mitosis (green) in mutant compared with WT. ( k ) Confocal microscope images of MEFs in prometaphase stained with antibodies against α-tubulin (α-tub., red) and γ-tubulin (γ-tub., green). Hoechst stains chromosomes (blue). Note the increased centrosome numbers (γ-tubulin staining) in the mutant compared with WT. Scale bar, 2 μm. ( i ) Quantification of multipolar spindles in experiment k . Data represents s.e.m. of three independent experiments, counting at least 5,000 MEFs per experiment ( P =0.011, Student’s t -test). Full size image To follow the fate of individual cells we performed time-lapse imaging studies. Wild-type MEFs underwent mitosis in an average of 60–70 min, whereas Wdr62 mutant MEFs stayed in mitosis for an average of 90–100 minutes with some mutant cells in mitosis for more than 400 min ( Fig. 4f–j , Supplementary Movies 1–3 ), consistent with a mitotic arrest phenotype. In addition, a significant number of mutant cells exhibited delayed mitotic progression and subsequently died during mitosis (red arrowheads in Fig. 4h,j , Supplementary Movie 3 ), suggesting that mitotic delay eventually leads to cell death in the Wdr62 depleted MEFs. We also observed a significant increase in number of mutant cells that aborted cell division ( Fig. 4g,j , Supplementary Movie 2 ). Aborted cell division can result in supernumerary centrosomes [19] . Indeed, there was a significant increase of mutant MEFs with multipolar spindles with colocalized γ-tubulin and centrin compared with wild type ( Fig. 4k,l and Supplementary Fig. 6b ). These quantitative and dynamic analyses of MEFs indicated that Wdr62 is required for mitotic progression, and the loss of Wdr62 function causes mitotic delay that ultimately results in cell death of a portion of mutant cells. Wdr62 depletion causes SAC activation The mitotic arrest and cell death phenotypes in Wdr62 mutant NPCs ( Fig. 3 ) and MEFs ( Fig. 4 ) suggest the activation of the SAC [17] , [20] . We examined the expression of the kinetochore-associated checkpoint protein Mad2, which monitors the microtubule attachment on kinetochores [21] , [22] . In wild-type metaphase cells, Mad2 has left the kinetochores, however, this checkpoint protein remained present on the kinetochores of mutant cells in metaphase ( Fig. 5a,c ), including on unaligned chromosomes (white arrowheads and white box 1 in Fig. 5a ). We next monitored tension across sister kinetochores using the checkpoint protein BubR1 (refs 21 , 22 ). Indeed, the numbers of metaphase cells with BubR1 expression were significantly increased in mutant MEFs compared with control cells ( Fig. 5b,c ). Furthermore, there was a >4-fold increase in cells with unaligned or lagging chromosomes upon depletion of Wdr62 ( Fig. 5d,e ). Consistent with the association of Wdr62 with centrosomes and spindle microtubules ( Supplementary Fig. 5 ), these studies indicate that loss of Wdr62 functions compromises microtubule–kinetochore attachment and the tension across sister kinetochores, leading to the activation of the spindle checkpoint. 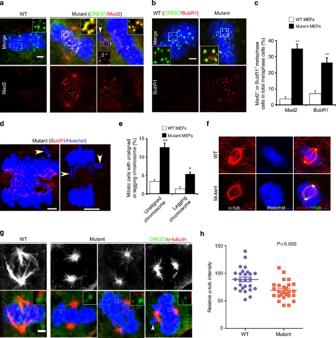Figure 5: Wdr62 regulates spindle assembly and its depletion activates the spindle checkpoint. (a,b) Wild-type and mutant MEFs at metaphase were co-stained for CREST (green), Mad2 (red ina) and BubR1 (red inb). Inserts show single focal planes of boxed regions. White arrowhead inapoints to unaligned chromosome. Scale bar, 2 μm. (c) Quantification of percentage of Mad2 or BubR1 positive metaphase cells out of the total metaphase cells inaandb, respectively. Data represent s.e.m. of three independent experiments, counting at least 50 metaphase cells per experiment (**P<0.01, Student’st-test). (d) Confocal microscope images of mutant cells at anaphase stained with BubR1. Hoechst stains nuclei (blue). White arrowheads mark unaligned or lagging chromosomes. Scale bars, 2.5 μm, 5 μm. (e) Quantification of percentage of mitotic cells with unaligned or lagging chromosomes. Data represent s.e.m. of three independent experiments, counting at least 50 metaphase or anaphase cells per experiment (**P<0.01, *P<0.05, Student’st-test). (f) Confocal microscope images of WT and mutant MEFs in metaphase stained with antibodies against α-tubulin (red) and γ-tubulin (green). Hoechst stains nuclei (blue). Scale bar, 2 μm. (g) Confocal microscope images of MEFs incubated at 4 °C for 40 min and co-stained with antibodies against α-tubulin (red) and CREST (green). Hoechst stains nuclei (blue). Inserts show single focal planes of boxed regions. White arrowhead points to unaligned chromosome. Scale bar, 2 μm. (h) The relative intensity of α-tubulin in wild-type (blue) and mutant (red) cells within metaphase spindle was measured using quantitative fluorescence imaging. Data represent s.e.m. of >25 cells for each genotype (P<0.002, Student’st-test). Figure 5: Wdr62 regulates spindle assembly and its depletion activates the spindle checkpoint. ( a , b ) Wild-type and mutant MEFs at metaphase were co-stained for CREST (green), Mad2 (red in a ) and BubR1 (red in b ). Inserts show single focal planes of boxed regions. White arrowhead in a points to unaligned chromosome. Scale bar, 2 μm. ( c ) Quantification of percentage of Mad2 or BubR1 positive metaphase cells out of the total metaphase cells in a and b , respectively. Data represent s.e.m. of three independent experiments, counting at least 50 metaphase cells per experiment (** P <0.01, Student’s t -test). ( d ) Confocal microscope images of mutant cells at anaphase stained with BubR1. Hoechst stains nuclei (blue). White arrowheads mark unaligned or lagging chromosomes. Scale bars, 2.5 μm, 5 μm. ( e ) Quantification of percentage of mitotic cells with unaligned or lagging chromosomes. Data represent s.e.m. of three independent experiments, counting at least 50 metaphase or anaphase cells per experiment (** P <0.01, * P <0.05, Student’s t -test). ( f ) Confocal microscope images of WT and mutant MEFs in metaphase stained with antibodies against α-tubulin (red) and γ-tubulin (green). Hoechst stains nuclei (blue). Scale bar, 2 μm. ( g ) Confocal microscope images of MEFs incubated at 4 °C for 40 min and co-stained with antibodies against α-tubulin (red) and CREST (green). Hoechst stains nuclei (blue). Inserts show single focal planes of boxed regions. White arrowhead points to unaligned chromosome. Scale bar, 2 μm. ( h ) The relative intensity of α-tubulin in wild-type (blue) and mutant (red) cells within metaphase spindle was measured using quantitative fluorescence imaging. Data represent s.e.m. of >25 cells for each genotype ( P <0.002, Student’s t -test). Full size image To understand why Wdr62 depletion results in defective microtubule–kinetochore attachment and SAC activation, we examined the centrosomes because spindle assembly depends on centrosome biogenesis and functions [23] , and several MCPH proteins are implicated in centriole biogenesis or centrosome maturation [16] , [24] , [25] . In Wdr62 mutant MEFs, proteins involved in centrosome biogenesis exhibited normal expression patterns, including ninein (a marker for mature mother centrioles), centrin (a marker of individual centrioles) and PCM (pericentriolar material) markers (γ-tubulin, Pericentrin and PCM-1) ( Supplementary Fig. 6a ). We next examined the spindle morphology and found that a small number of mutant mitotic cells exhibited aberrant spindles with reduced microtubule density, as indicated by total α-tubulin immunofluorescence intensity, compared with control ( Fig. 5f ), suggesting that spindle integrity may be compromised in mutant cells. Under conditions that destabilize microtubules such as cold, less stable microtubules undergo depolymerization and relatively stable microtubule populations, such as kinetochore fibres, remain intact [26] . In wild-type MEFs following a short exposure to cold, the kinetochore microtubule fibre subpopulation remains relatively intact with a bipolar shape ( Fig. 5g ). In contrast, in mutant cells there was a reduction in the number, length and density of α-tubulin staining of kinetochore microtubules ( Fig. 5g,h shows quantification of α-tubulin staining in metaphase cells). Thus, spindle assembly and function are compromised in Wdr62 deficient cells, and this could explain the SAC activation and mitotic progression delay of mutant cells. Wdr62 depletion delays mitotic progression of NPCs in vivo Given that our Wdr62 deficient line is hypomorphic ( Fig. 1a–c ) and our mechanistic analysis of mitotic defects was largely gained from studies in MEFs ( Figs 4 and 5 ), we used siRNA/shRNA as independent approaches to knockdown Wdr62 functions in the developing brain ( Supplementary Fig. 7a,b ). Co-electroporation of Wdr62 siRNA with H2BGFP plasmids and live imaging of brain slice cultures viewed from the ventricular surface allowed us to follow individual NPCs, and examine Wdr62 cell-autonomous roles during mitotic progression ( Supplementary Fig. 7 and Supplementary Movie 4 ) [27] , [28] . Consistent with the increased mitotic delay observed in mutant MEFs ( Fig. 4 ), knockdown of Wd62 function significantly delayed the mitotic progression of individual NPCs compared with control siRNA treated cells ( Fig. 6a,b , Supplementary Movies 5–8 ). Thus, these data suggest that Wdr62 regulates mitotic progression and its depletion results in mitotic delay in vivo . 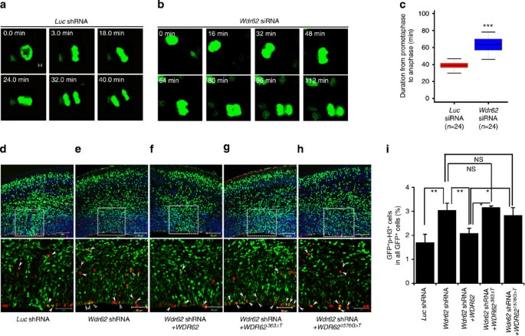Figure 6:Wdr62depletion delays mitotic progression of neural progenitor cellsin vivo. (a,b) Still images from time-lapse movies of E14.5 dividing cortical neural progenitor cells 30 h afterin uteroelectroporation with luciferase siRNA plus pCAG-H2BGFP plasmids (a) orWdr62siRNA plus pCAG-H2BGFP plasmids (b). Images were taken every 4 min. Scale bars, 2 μm. (c) Quantification of the duration from prometaphase to anaphase of mitotic cells from experimenta,b. Data are expressed as s.e.m. of three independent experiments, counting 24 individual dividing cells per experiment (***P<0.005, Student’st-test). (d–h) 60 h afterin uteroelectroporation of indicated constructs together with pCAG-H2BGFP plasmids into E13.5 brains, cerebral cortex sections were stained with GFP (green) and p-H3 (red). (i) Quantification of percentage of GFP/p-H3 double positive cells out of total GFP-positive cells from experimentse–id–h. All data represent mean±s.e.m. of three independent experiments (two embryos per group per experiment; *P<0.05; **P<0.01; NS, not significant one-way analysis of variance test). Figure 6: Wdr62 depletion delays mitotic progression of neural progenitor cells in vivo . ( a , b ) Still images from time-lapse movies of E14.5 dividing cortical neural progenitor cells 30 h after in utero electroporation with luciferase siRNA plus pCAG-H2BGFP plasmids ( a ) or Wdr62 siRNA plus pCAG-H2BGFP plasmids ( b ). Images were taken every 4 min. Scale bars, 2 μm. ( c ) Quantification of the duration from prometaphase to anaphase of mitotic cells from experiment a , b . Data are expressed as s.e.m. of three independent experiments, counting 24 individual dividing cells per experiment (*** P <0.005, Student’s t -test). ( d – h ) 60 h after in utero electroporation of indicated constructs together with pCAG-H2BGFP plasmids into E13.5 brains, cerebral cortex sections were stained with GFP (green) and p-H3 (red). ( i ) Quantification of percentage of GFP/p-H3 double positive cells out of total GFP-positive cells from experiments e – i d–h . All data represent mean±s.e.m. of three independent experiments (two embryos per group per experiment; * P <0.05; ** P <0.01; NS, not significant one-way analysis of variance test). Full size image As the basis for an assay for structure-function studies of Wdr62 disease alleles, we tested whether expression of full-length human WDR62 could rescue the mitotic progression defect of Wdr62 deficient NPCs in mice. Using in utero electroporation, knockdown of Wdr62 significantly delayed mitotic progression of NPCs as assessed by increased numbers of p-H3-positive cells ( Fig. 6d,e ), consistent with the analysis of Wdr62 mutants ( Fig. 3a–g ). Introduction of human WDR62 , which is resistant to mouse Wdr62 shRNA knockdown, significantly rescued this mitotic progression defect ( Fig. 6d–f,i ). These studies independently confirm that the mitotic defect in Wdr62 mutant NPCs is due to the loss of Wdr62 and provide a functional assay for WDR62 disease alleles. We then focused on two individual nonsense mutant alleles WDR62 363ΔT (ref. 11 ) and WDR62 1576G>T (ref. 29 ), which are predicted to generate N-terminal truncated proteins of 121 and 525 aa, respectively. In contrast to wild-type WDR62, neither WDR62 363ΔT nor WDR62 1576G>T could rescue the mitotic progression defect of Wdr62 deficient NPCs ( Fig. 6g–i ), suggesting that these disease alleles could disrupt the mitotic progression of NPCs during brain development. Wdr62 associates with and regulates Aurora A To understand the molecular mechanisms by which Wdr62 regulates mitotic progression, we next tested whether Wdr62 physically interacts with factors involved in mitotic spindle assembly. After screening a set of Wdr62 associated proteins using co-immunoprecipitation assays, we found that endogenous Wdr62 specifically interacts with two major regulators of spindle assembly, Aurora A kinase and Tpx2 ( Fig. 7a , Supplementary Fig. 8a ) [30] , [31] . Pull-down experiments verified the association between Wdr62 with Aurora A and with Tpx2 ( Fig. 7b,c , Supplementary Fig. 10b ). To determine the region of interaction within the Wdr62 protein, a series of N- and C-terminal deletions of Wdr62 were generated. Mapping studies using these deletion constructs showed that Aurora A and Tpx2 interact with the middle region (621–1,138 aa) of Wdr62 ( Fig. 7d,e , Supplementary Fig. 10c–e ). Together, these studies suggest that Wdr62 associates with Aurora A and Tpx2. 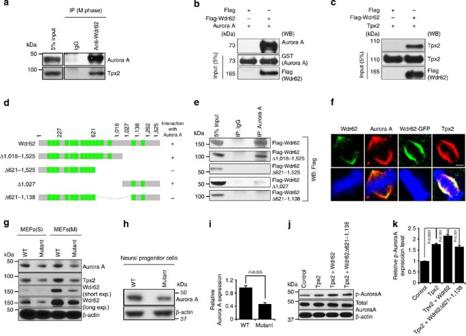Figure 7: Wdr62 interacts with and regulates Aurora A protein levels and activities. (a) Endogenous Wdr62 protein was immunoprecipitated with anti-Wdr62 antibodies from 293T cells arrested in M phase. Coimmunoprecipitated proteins were analysed by western blot with indicated antibodies. (b,c) Direct interaction between Wdr62 and Aurora A or Tpx2 was assessed by Flag pull-down using purified Flag-Wdr62 protein and recombinant GST-Aurora A protein (b) or HA-Tpx2 protein (c). (d) Schematic summary of the interactions between Aurora A with full-lengthWdr62or variousWdr62deletion constructs. (e) Total lysates from M phase 293T cells transfected with flag-taggedWdr62or variousWdr62deletion constructs, followed by immunoprecipitation with anti-Aurora A antibody, and western blot analysis performed with anti-Flag antibody. (f) Confocal microscope images of wild-type or Wdr62-GFP transfected MEFs in metaphase co-labelled with antibodies against Wdr62 (green)/Aurora A (red) or GFP (green)/Tpx2 (red). Hoechst stains chromosomes (blue). (g,h) Western blot analyses of Aurora A expression in S phase or M phase arrested MEFs (g) and isolated neural progenitor cells from E17.5 cerebral cortex (h) from wild-type and mutant embryos. β-actin serves as loading control. (i) Quantification of Aurora A protein levels from experimenth; s.e.m. from three independent experiments (two embryos per group per experiment,P<0.005, Student’st-test). (j) Wdr62 enhances Tpx2-mediated activation of Aurora A (phosphorylated Aurora A). Different constructs as indicated were transfected into HeLa cells, and 24 h post transfection, 100 ng ml−1Nocodazole was added to cultured cells for 14–16 h before western blot analysis. (k) Quantification of expression of p-Aurora A versus total Aurora A using data from experimentj. Data expressed as s.e.m. of three independent experiments,P<0.001 (Student’st-test). Figure 7: Wdr62 interacts with and regulates Aurora A protein levels and activities. ( a ) Endogenous Wdr62 protein was immunoprecipitated with anti-Wdr62 antibodies from 293T cells arrested in M phase. Coimmunoprecipitated proteins were analysed by western blot with indicated antibodies. ( b , c ) Direct interaction between Wdr62 and Aurora A or Tpx2 was assessed by Flag pull-down using purified Flag-Wdr62 protein and recombinant GST-Aurora A protein ( b ) or HA-Tpx2 protein ( c ). ( d ) Schematic summary of the interactions between Aurora A with full-length Wdr62 or various Wdr62 deletion constructs. ( e ) Total lysates from M phase 293T cells transfected with flag-tagged Wdr62 or various Wdr62 deletion constructs, followed by immunoprecipitation with anti-Aurora A antibody, and western blot analysis performed with anti-Flag antibody. ( f ) Confocal microscope images of wild-type or Wdr62-GFP transfected MEFs in metaphase co-labelled with antibodies against Wdr62 (green)/Aurora A (red) or GFP (green)/Tpx2 (red). Hoechst stains chromosomes (blue). ( g , h ) Western blot analyses of Aurora A expression in S phase or M phase arrested MEFs ( g ) and isolated neural progenitor cells from E17.5 cerebral cortex ( h ) from wild-type and mutant embryos. β-actin serves as loading control. ( i ) Quantification of Aurora A protein levels from experiment h ; s.e.m. from three independent experiments (two embryos per group per experiment, P <0.005, Student’s t -test). ( j ) Wdr62 enhances Tpx2-mediated activation of Aurora A (phosphorylated Aurora A). Different constructs as indicated were transfected into HeLa cells, and 24 h post transfection, 100 ng ml −1 Nocodazole was added to cultured cells for 14–16 h before western blot analysis. ( k ) Quantification of expression of p-Aurora A versus total Aurora A using data from experiment j . Data expressed as s.e.m. of three independent experiments, P <0.001 (Student’s t -test). Full size image To explore the mechanistic basis of the interaction between Wdr62 and Aurora A, we first examined the localization of Wdr62 and Aurora A/Tpx2. Wdr62 co-localizes with Aurora A and Tpx2 during different phases of mitosis ( Fig. 7f ). Aurora A and Tpx2 show normal localization in Wdr62 mutant MEFs, however, the level of Aurora A appeared to be decreased in mutant MEFs ( Supplementary Fig. 8b ). To explore this latter point further, we examined the expression levels of Aurora A, and found that it was significantly downregulated in mutant MEFs ( Fig. 7g , Supplementary Fig. 10f–h ) and isolated NPCs ( Fig. 7h,i , Supplementary Fig. 10i,j ). Furthermore, Wdr62 enhances Tpx2-mediated Aurora A activation ( Fig. 7j,k , Supplementary Fig. 8d,e ), although Wdr62 itself is not sufficient to activate Aurora A in vitro ( Supplementary Fig. 8c ). In contrast to full-length Wdr62, Wdr62Δ621–1,138 does not activate Aurora A kinase activity ( Fig. 7j,k , Supplementary Fig. 10k ), likely due to its loss of interaction with Aurora A. Together, these studies suggest that Wdr62 positively regulates Aurora A protein levels and kinase activities in the presence of Tpx2. Wdr62 genetically interacts with Aurora A to regulate mitosis The observations above suggest that Wdr62 could functionally interact with Aurora A to regulate mitotic progression. This is consistent with mitotic arrest phenotype observed in Wdr62 ( Fig. 4 ) and in Aurora A mutant MEFs [32] . To test this idea genetically, we crossed Wdr62 +/− mice with Aurora A +/− mice. Compound heterozygous animals were observed at a much lower frequency (7%) than Mendelian expectation of 25%. Of those double heterozygous animals that survived, many were much smaller compared with single heterozygotes ( Fig. 8a ). Examination of the cerebral cortex of double heterozygous P2 pups revealed significantly increased p-H3 staining ( Fig. 8b–d ) and reduced Pax6 positive NSCs ( Fig. 8b,c,e ), similar to that seen in Wdr62 mutant cortex ( Figs 2 and 3 ), suggesting mitotic progression delay of NPCs in double heterozygous animals. These data indicate that Wdr62 and Aurora A genetically interact to regulate mitotic progression of NPCs. 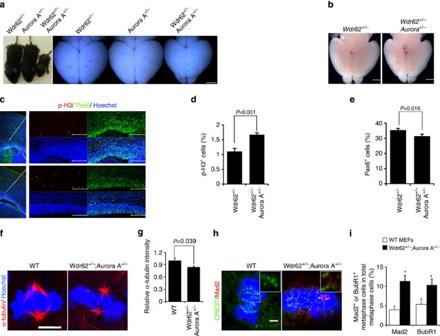Figure 8: Wdr62 genetically interacts with Aurora A to regulate mitotic progression and brain size. (a) P14 littermates showing overall body and brain size ofWdr62+/−heterozygote,Aurora A+/−heterozygote andWdr62+/−Aurora A+/−double heterozygote. Scale bar, 1.2 cm. (b,c) P2 brains and confocal micrographs of coronal sections fromWdr62+/−(upper panel) orWdr62+/−Aurora A+/−(lower panel) cerebral cortex stained with antibodies against phospho-histone H3 (p-H3) (red) and Pax6 (green). Hoechst stains nuclei (blue). Scale bars, 1 cm, 100 μm. (d,e) Quantification of p-H3 positive cells (d) and Pax6 positive cells (e) from experimentc. All data represent mean±s.e.m. of three independent experiments (two embryos per group per experiment,P=0.001 (d); 0.016 (e) (Student’st-test). (f) Confocal microscope images of MEFs incubated at 4 °C for 40 min and co-stained with antibodies against α-tubulin (red). Hoechst stains nuclei (blue). Scale bar, 5 μm. (g) The relative intensity of α-tubulin within metaphase spindle was measured using quantitative fluorescence imaging from experimentf. Data represent s.e.m. of more than 20 cells for each genotype (P=0.039, Student’st-test). (h) Wild-type and double heterozygous MEFs at metaphase were co-stained for CREST (green), Mad2 (red). Inserts show single focal planes of boxed regions. Scale bar, 2 μm. (i) Quantification of percentage of Mad2 or BubR1 positive metaphase cells out of the total metaphase cells. Data represent s.e.m. of three independent experiments, counting at least 25 metaphase cells per experiment (*P<0.05, Student’st-test). Figure 8: Wdr62 genetically interacts with Aurora A to regulate mitotic progression and brain size. ( a ) P14 littermates showing overall body and brain size of Wdr62 +/− heterozygote, Aurora A +/− heterozygote and Wdr62 +/− Aurora A +/− double heterozygote. Scale bar, 1.2 cm. ( b , c ) P2 brains and confocal micrographs of coronal sections from Wdr62 +/− (upper panel) or Wdr62 +/− Aurora A +/− (lower panel) cerebral cortex stained with antibodies against phospho-histone H3 (p-H3) (red) and Pax6 (green). Hoechst stains nuclei (blue). Scale bars, 1 cm, 100 μm. ( d , e ) Quantification of p-H3 positive cells ( d ) and Pax6 positive cells ( e ) from experiment c . All data represent mean±s.e.m. of three independent experiments (two embryos per group per experiment, P =0.001 ( d ); 0.016 ( e ) (Student’s t -test). ( f ) Confocal microscope images of MEFs incubated at 4 °C for 40 min and co-stained with antibodies against α-tubulin (red). Hoechst stains nuclei (blue). Scale bar, 5 μm. ( g ) The relative intensity of α-tubulin within metaphase spindle was measured using quantitative fluorescence imaging from experiment f . Data represent s.e.m. of more than 20 cells for each genotype ( P =0.039, Student’s t -test). ( h ) Wild-type and double heterozygous MEFs at metaphase were co-stained for CREST (green), Mad2 (red). Inserts show single focal planes of boxed regions. Scale bar, 2 μm. ( i ) Quantification of percentage of Mad2 or BubR1 positive metaphase cells out of the total metaphase cells. Data represent s.e.m. of three independent experiments, counting at least 25 metaphase cells per experiment (* P <0.05, Student’s t -test). Full size image To dissect the underlying causes of this mitotic defect of double heterozygous mice, we examined MEFs and found that spindle stability is significantly altered in MEFs from double heterozygous animals compared with controls ( Fig. 8f,g ). Consistently, there is significantly increased numbers of cells wherein the metaphase chromosomes show the presence of checkpoint protein Mad2 and BubR1 ( Fig. 8h,i ), suggesting SAC activation in the double heterozygous MEFs compared with controls. These phenotypes of altered spindle stability and SAC activation in double heterozygous MEFs mimic the main cellular phenotypes of Wdr62 deficient MEFs ( Fig. 5a–c,g,h ), indicating that Aurora A mediates, at least in part, the mitotic functions of Wdr62 at the cellular level. The data presented here suggest that centrosomal protein Wdr62 regulates mitotic progression of NPCs, loss of which results in NPC mitotic delay, cell death and smaller brains in mice. This mitotic function of Wdr62 in brain development is supported by our mouse genetic studies as well as the live imaging analysis from brain slices and cultured MEFs. A recent study from Bogoyevitch et al. [33] using Wdr62 siRNA suggested that Wdr62 regulates NPC cell cycle exit, proliferation capacity and spindle orientation. However, we did not detect significant changes of cell cycle exit or spindle orientation ( Supplementary Fig. 9 ) in our Wdr62 deficient mouse model, which could be due to different approaches used in these two studies or residual Wdr62 protein in our hypomorphic mutant. We show that Wdr62 regulates spindle stability in Wdr62 deficient MEFs, consistent with results by Bogoyevitch et al. in HeLa cells. Our study extends an understanding by demonstrating that Wdr62 deficient cells have a functional deficiency of spindles which results in SAC activation, and leads to mitotic arrest and cell death of mutant cells. Our mechanistic studies further indicate that Wdr62 associates with and genetically interacts with spindle assembly factor Aurora A to regulate its mitotic functions. Together, these studies suggest that Wdr62 controls mitotic progression and cell survival of NPCs through, at least in part, regulation of Aurora A. Our live imaging analysis of MEFs suggests that mitotic arrest can lead to cell death; due to technical limitations we could not follow NPCs showing mitotic delay for a sufficient period to correlate with cell death in vivo . It is possible that Wdr62 independently regulates mitotic progression and cell death. In this scenario, Aurora A depletion could result in cell death through regulating alternative splicing, which precedes mitotic arrest [34] . Aurora A has multiple functions in cell cycle regulation, including centrosome separation [30] , [32] . It remains to be determined precisely which Aurora A functions are perturbed by Wdr62 insufficiency. Although several proteins involved in centrosome biogenesis exhibited normal expression pattern in mutant cells, this does not exclude an effect of Wdr62 deficiency on centrosome biogenesis. Moreover, we cannot rule out the possibility that Wdr62 functions through other proteins. For instance, it has been reported that WDR62 associates with JNK and mediates non-classical JNK activation [35] , [36] , which could contribute to the Wdr62 mutant phenotype. Current microcephaly gene studies have emphasized the roles of the MCPH proteins in diverse cellular processes. The predominant model invokes disrupted spindle orientation and defective symmetric/asymmetric division of NPCs [4] , [5] . Our studies of the Wdr62 mutant brains show that spindle orientation pattern is not disturbed in mutant NPCs of the cerebral cortex ( Supplementary Fig. 9 ) and differentiation is not induced prematurely, two phenotypes that would be expected if there were a disruption of symmetric/asymmetric cell division and coupled premature differentiation. Therefore, our studies suggest an alternative model in which disruption of mitotic progression and cell death of NPCs could be potential causes of human microcephaly. Our preliminary data indicate that wild-type human WDR62, but not disease alleles, can rescue the mitotic phenotype of Wdr62 deficiency. Further detailed studies on individual WDR62 disease alleles are required to understand the disease mechanisms of WDR62 associated malformations of cortical development. In addition to microcephaly, Wdr62 depletion results in reduction in body and organ size, first observed at E17.5 and extending into adulthood. Increased mitotic index was detected in the eye, heart and lung as early as E17.5 ( Supplementary Fig. 1 ). These results suggest that proportional dwarfism could be due to the disruption of mitotic progression of tissue progenitor cells throughout the body. Wdr62 mutant mice and other mouse strains SIGTR ES cell line AF0003 containing beta-galactosidase-neomycin resistance gene-trap vector (BayGenomics) inserted into the Wdr62 locus ( Fig. 1a ) was used by Mutant Mouse Regional Resource Center (MMRRC) to generate chimeric offspring. Chimeric offspring were mated to 129S1/SvImJ mice and progeny screened for the Wdr62 lacZ allele using genotyping primer set: Wdr62F, Wdr62R and Wdr62β-geoR as described in Supplementary Table 1 . The Aurora A floxed allele and CMV -Cre allele were supplied by Jackson Lab. All animals were handled according to protocols approved by the Institutional Animal Care and Use Committee (IACUC) at the University of Colorado Denver. For timed pregnant mating, noon of the day after mating was considered embryonic day 0.5 (E0.5). Analysis of mutant phenotype For RNA in situ hybridization, Wdr62 probe was amplified using the primers ( In situ -Wdr62F/R) listed in Supplementary Table 1 . The hybridization buffer is composed of 50% formamide, 5xSSC (pH=4.5), 50 μg ml −1 yeast tRNA, 1% SDS and 50 μg ml −1 heparin. Histological processing, TUNEL assay, immunohistochemical labelling of cryosections were performed using cerebral cortex sections from different stages of embryos as indicated in the figure and text. The primary antibodies are listed in Supplementary Table 2 . The secondary antibodies used were Alexa 488 and Alexa 555 conjugated to specific IgG types (Invitrogen Molecular Probes). All the experiments have been repeated at least three times, and representative images are shown in the individual figures. BrdU labelling and analysis E15.5, E16.5 or E17.5 pregnant mice were injected intraperitoneally with BrdU at 25 μg g −1 of body weight. The animals were sacrificed 1 or 24 h after the injection. The brains were dissected out and fixed in 4% paraformaldehyde overnight. Subsequently, the brains were stored in 30% sucrose for 16 h and embedded in the O.C.T. solution. Anti-Wdr62 antibody generation and purification The 1,524 bp fragment indicated in Fig. 1a (which encodes the C-terminal end of Wdr62) was amplified using the GSTWdr62F/R primers listed in Supplementary Table 1 . GSTWdr62 construct and fusion protein were generated according to standard molecular methods. Covance Inc. generated and purified the antibody using GSTwdr62 protein as the antigen. MEF isolation and time-lapse imaging MEFs were isolated from E15.5 embryos as described and cultured in Dulbecco's Modified Eagle's Medium (DMEM) with 10% fetal bovine serum and 0.075% penicillin/streptomycin. Time-lapse images were acquired using a Zeiss LSM510 confocal microscope using a heated chamber and 5% CO 2 . Images were captured at 10-minute intervals using a × 10 PlanApo lens. Cell culture and synchronization HeLa cells and 293T cells were obtained from the American Type Culture Collection (ATCC) and cultured in DMEM (Invitrogen) supplemented with 10% FBS. To obtain S-phase arrested cells, 293T cells were incubated with 1 mM hydroxyurea for 16 h. To arrest cells in M-phase, 100 ng ml −1 nocodazole was added to the 293T cells for 16 h before the collection. To obtain M-phase arrested MEFs, wild-type and mutant MEFs at passage 3 were synchronized at the G1/S boundary by blocking with 2.5 mM thymidine for 16 h, released in the fresh DMEM (10% FBS) medium for 8 h, and then blocked for 14 h with 2.5 mM thymidine. Cells were then released into DMEM (10% FBS) medium containing 100 ng ml −1 nocodazole for 24 h to obtain a relatively synchronized population of cells arrested in mitosis. Purification of Flag-Wdr62 protein and in vitro kinase assay Flag-Wdr62 plasmids were transfected into 293T cells and selected by puromycin (5 μg ml −1 ) to generate stable cell lines. Crude lysate was collected in the lysis buffer (20 mM Tris–HCl (pH 7.5), 137 mM NaCl, 1 mM EDTA, 1.5 mM MgCl 2 , 10% Glycerol, 0.2% Triton X-100). To purify the Flag-Wdr62 proteins, cytoplasmic extract was incubated with anti-Flag M2 affinity resin (Sigma). After extensive washing with wash buffer (20 mM Tris–HCl (pH 7.5), 0.8 M NaCl), the affinity column was eluted with 400 μg ml −1 Flag peptide. Proteins were further separated with Superose 6 gel filtration chromatography. Fractions were examined by SDS–PAGE analysis, and fractions containing Wdr62 protein were combined and concentrated with Millipore Amicon Ultra (100 K). Purified proteins were snap-frozen in liquid nitrogen and stored at −80 °C. For in vitro kinase assay, purified Flag-Wdr62 proteins or commercially available Tpx2 proteins (SignalChem, cat# T40-30H-20) and Aurora A proteins (SignalChem, cat# A28-18G) were incubated with 25 μM ATP and 4 uCi γ-[ 32 P]-ATP in 20 ul of reaction mixture containing 50 mM Tris–HCl, pH 7.5, 25 mM NaCl, 1 mM DTT, and 10 mM MgCl 2 . After reacting for 15 min at 30 °C, the protein-loading buffer was added and boiled for 5 min for SDS–PAGE gel separation. Gels were autoradiographied with Storm 840 (Molecular Dynamics). Pull-down and immunoprecipitation Purified Flag-Wdr62 proteins were incubated with anti-Flag M2 affinity resin (Sigma). 5 μg of Tpx2 proteins (SignalChem, cat# T40-30H-20) or Aurora A proteins (SignalChem, cat# A28-18G) were added to the beads in the pull-down buffer containing 20 mM Hepes (pH 7.9], 150 mM NaCl, 0.5 mM EDTA, 10% Glycerol, 0.1% Triton X-100 and 1 mM DTT). The beads were rocked at 4 °C for 2 h and washed with 5 × 800 μl of pull-down buffer before assaying by Western blot. For immunoprecipitation, cells were lysed in lysis buffer (50 mM Tris–HCl (pH7.4), 150 mM NaCl, 1 mM EDTA, 1% Triton X-100 and 1 tablet protease inhibitor (Roche) per 10 ml). Cell debris was pelleted at 12,500 r.p.m. for 10 min at 4 °C and the supernatant was incubated with primary antibodies overnight at 4 °C. The lysates with antibodies were incubated with Protein A/G Sepharose beads for 2 h, followed by washing of the immunoprecipitates three times with lysis buffer and elution of bound proteins in SDS–PAGE sampling buffer at 100 °C for 10 min. Western blots were performed using the antibodies described in Supplementary Table 2 . NPC isolation The cerebral cortex was cut into small pieces of about 1 mm, and then digested with papain (10 units ml −1 ) (Worthington LS 03126) enzyme solution at 37 °C for 30 min. The tissue was moved sequentially from high concentration trypsin inhibitor (0.1 g ml −1 ), to low concentration trypsin inhibitor (0.01 g ml −1 ), and to serum-free medium (Basal medium with B27). The tissue was triturated gently 10 to 20 times, which resulted in the dissociation of the tissues into a single-cell suspension. The cells were plated onto poly- D -lysine/laminin coated plates. In utero electroporation DNA constructs including pCAG-H2BGFP, Wdr62 shRNA, human WDR62 plasmids or Wdr62 siRNA plus 0.5% Fast Green (Sigma) were injected into the lateral ventricle of E13.5 wild-type embryos followed by electroporation using an ECM 830 electroporator (BTX) with four 100 ms pulses separated by 100 ms intervals at 35 V. To improve retention of the pregnancy, we avoided plasmid injection and electroporation of the two embryos next to the ovaries and the two embryos next to upper vagina. The ON-Target plus SMART pool of Wdr62 siRNAs was purchased from Dharmcon. In utero development was allowed to continue for 24 h (or as indicated), then the embryos were dissected and cortical region was processed for immunohistochemistry or time-lapse imaging. How to cite this article: Chen, J.-F. et al. Microcephaly disease gene Wdr62 regulates mitotic progression of embryonic neural stem cells and brain size. Nat. Commun. 5:3885 doi: 10.1038/ncomms4885 (2014).